Reduced time as a unified parameter determining fixity and free recovery of shape memory polymers Shape memory polymers are at the forefront of recent materials research. Although the basic concept has been known for decades, recent advances in the research of shape memory polymers demand a unified approach to predict the shape memory performance under different thermo-temporal conditions. Here we report such an approach to predict the shape fixity and free recovery of thermo-rheologically simple shape memory polymers. The results show that the influence of programming conditions to free recovery can be unified by a reduced programming time that uniquely determines shape fixity, which consequently uniquely determines the shape recovery with a reduced recovery time. Furthermore, using the time–temperature superposition principle, shape recoveries under different thermo-temporal conditions can be extracted from the shape recovery under the reduced recovery time. Finally, a shape memory performance map is constructed based on a few simple standard polymer rheology tests to characterize the shape memory performance of the polymer. The concept of shape memory polymers (SMPs) [1] , [2] , [3] , [4] , [5] , [6] has been known for decades [7] , [8] , [9] , [10] , [11] , [12] , [13] . In general, the polymer’s shape memory (SM) effect is described and evaluated in a thermo-temporal SM cycle, where the SMP is firstly deformed at a high temperature (usually above the glass transition or melting point) and subsequently frozen upon cooling to fix the programmed temporary shape. When an environmental stimulus is applied, the SMP could either provide recovery stresses or return to their permanent shapes, depending on whether or not the external loads still exist, namely the constrained or free recovery condition [14] , [15] , [16] , [17] , [18] , [19] , [20] , [21] , [22] , [23] , [24] , [25] , [26] , [27] , [28] , [29] , [30] . Since SMPs can sense the environmental changes and then take reactions in a predetermined sequence with deformation, they are considered as a promising alternative for the future’s spontaneous shape changing and tunable components in various applications such as microelectromechanical systems, surface patterning, biomedical devices, aerospace deployable structures and morphing structures [31] , [32] , [33] , [34] , [35] , [36] , [37] , [38] , [39] . An SM cycle typically involves a programming step and a recovery step. The programming step includes thermo-temporal conditions such as programming (loading) temperature, loading rate, holding time after loading, cooling rates and shape fixing temperature; the recovery step includes heating rates, recovery temperature and holding time at the recovery temperature. The performance of a thermally triggered SMPs is typically quantified by shape fixity, shape recovery rate and ratio, shape recovery stiffness and stress, and so on [40] , [41] , [42] , [43] , [44] , [45] , [46] , [47] , [48] , [49] , [50] . Previous experimental work revealed complicated dependency of the SM performance on thermo-temporal conditions in an SM cycle. For example, the recovery of SMPs programmed under the same conditions strongly depends on the recovery temperature and heating rate in the recovery step [43] , [46] , [47] , [48] , [49] , [50] , [51] , [52] ; in addition, the programming temperature has been shown to affect significantly the free recovery behaviour for SMPs under the same thermo-temporal recovery conditions [31] , [53] , [54] , [55] , [56] , [57] . To date, because the recovery behaviour of an SMP depends on the aforementioned multiple thermo-temporal input parameters, there is no clear understanding how these input parameters can affect the SM performance individually or collectively. Such complicated dependency also hinders the development of SMP applications from the material and product design point of view. Therefore, a method that can unify the thermo-temporal conditions and quantify the SM performance is highly desirable by the community. In addition, it is important that the parameters in this method can be obtained by a few simple or standard experiments. This paper studies the shape fixity and free recovery of thermo-rheologically simple SMPs that utilize glass transition to achieve the SM effect, with the goal of unravelling the complicated dependency of SM performance on thermo-temporal conditions of this type of SMPs. Experimental observations firstly reveal the influence of programming temperature ( T d ), holding time at T d and shape recovery temperature T r on the free shape recovery behaviour of an acrylate-based SMP material. An analytical solution based on the one-dimensional multi-branch rheological model is then applied to unravel the complicated dependences of the polymer SM effect on both programming and recovery conditions. The results show that the effect of programming conditions can be unified by a reduced programming time that uniquely determines shape fixity, which consequently uniquely determines the shape recovery with a reduced recovery time. In addition, the free recovery behaviours follow the time-temperature superposition principle. Finally, a SM performance map (SMP map) is constructed as a unified approach to characterize the SM performance. The SMP map can be constructed by using parameters obtained from stress relaxation experiments at different temperatures and a DMA test, which are standard rheological tests in polymer physics. Thermo-rheological description of SMPs As well known in polymer physics, the thermomechanical properties of a thermo-rheologically simple polymer can be described by a multi-branch rheological model, shown in Fig. 1 . The model consists of one equilibrium branch and several thermoviscoelastic nonequilibrium branches (number of n ) to represent the multiple relaxation processes of the polymer. 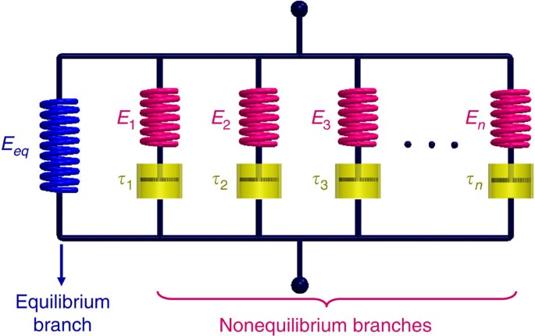Figure 1: Multi-branch rheological model. 1D rheological representation of the multi-branch model. By applying the Boltzmann’s superposition principle [58] , the total stress σ ( t ) of the model is: Figure 1: Multi-branch rheological model. 1D rheological representation of the multi-branch model. Full size image with to describe the elastic strain evolution in each nonequilibrium branches. In Equations 1 and 2, e m ( t ) is the total strain. E eq and E i are the elastic moduli in the equilibrium and nonequilibrium branches, respectively. τ i ( T ) denotes the temperature-dependent relaxation time in the dashpots, which follows the time–temperature superposition principle (TTSP) [58] and serves as a cornerstone in transforming the polymer behaviours between short-time range at high temperature and long-time range at low temperature. After determining the model parameters by using the stress relaxation master curve of an acrylate crosslinking SMP (shown in Supplementary Note 1 ), the model shows the capability of capturing the temperature-dependent free recovery behaviour of SMP, and therefore is validated as an effective tool to assist the subsequent theoretical discussions [44] , [45] , [47] . Experimental observations on shape fixity and recovery As shown in Fig. 2a , we define a representative SM cycle as the following: In the programming step, the SMP is stretched to a target strain e max (20%) with a constant loading rate (0.01 s −1 ) at the programming temperature T d , followed by a specified holding time at T d before being cooled to the shape-fixing temperature T L (20 °C) at a rate of q (2.5 °C min −1 ). Once T L is reached, the specimen is held for 1 hour and then the tensile force is removed. In the free recovery step, the temperature is increased to the recovery temperature T r at the same rate of cooling and subsequently stabilized for another 50 min. 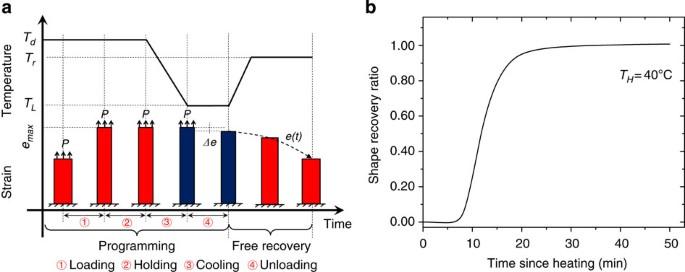Figure 2: A typical SM cycle. (a) A schematic illustration of the thermomechanical history of the programming and free recovery process in an SM cycle. (b) A typical free recovery curve as a function of time. Figure 2: A typical SM cycle. ( a ) A schematic illustration of the thermomechanical history of the programming and free recovery process in an SM cycle. ( b ) A typical free recovery curve as a function of time. Full size image As shown in Fig. 2a , usually there is a small bouncing back of the material upon unloading (step 4), which causes some loss in shape fixing. Therefore, the shape fixity R f is defined as [59] : where e r is the strain measured at the start of the free recovery process with e r = e max −Δ e and e ( t ) is the time-dependent strain measured at the free recovery process. The shape recovery is a function of time (and temperature), as shown in Fig. 2b for a typical case. Thus, the shape recovery ratio R r is defined as [59] : Several groups of experiments were conducted to study the dependency of shape fixity and recovery on the programming and recovery conditions. In the first experimental investigation, the SMP specimens were respectively programmed at 11 different temperatures ( T d is evenly distributed from 25–50 °C) and recovered at 40 °C ( T r =40 °C). The shape fixities and the shape recovery times corresponding to the 95% shape recovery ratio ( t 0.95 ) are plotted as a function of programming temperature in Fig. 3a . The measured shape recovery ratio is plotted as a function of heating time in Fig. 3b . 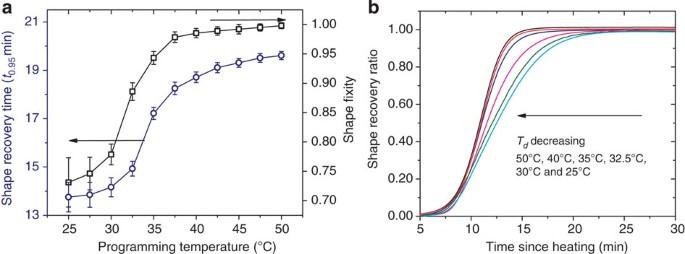Figure 3: Effects of programming temperatures on shape fixity and shape recovery. (a) Shape fix ratio and shape recovery time (t0.95) as a function of programming temperature (evenly distributed from 25–50 °C) (b) Shape recovery ratio as a function of heating time. Figure 3a,b shows that a lower programming temperature has two effects: On the one hand, it results in a faster shape recovery rate. This phenomenon is referred as temperature memory effect of SMPs under free recovery condition [55] , [57] , [60] . On the other hand, however, it leads to lower shape fixity, indicating that a large portion of the programmed deformation is recovered right after unloading. Such a sudden spring back at low programming temperatures would cause some instabilities for the length measurement in the adopt machine (DMA, TA Instruments, Model Q800), which subsequently results in the elevated experimental uncertainties as shown in Fig. 3a . Figure 3: Effects of programming temperatures on shape fixity and shape recovery. ( a ) Shape fix ratio and shape recovery time ( t 0.95 ) as a function of programming temperature (evenly distributed from 25–50 °C) ( b ) Shape recovery ratio as a function of heating time. 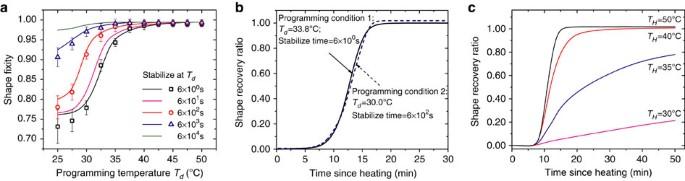Figure 4: Effects of holding time on Shape fixity and shape recovery. (a) Shape fixity as a function of programming temperature (Td) and holding time atTd. Note: dots denote the experimental results and solid lines denote simulation results the low temperatureTLis always 20 °C in all the experimental cases. (b) Shape recovery behaviour of SMPs experienced by two programming conditions that achieve the same shape fix ratio (90%). (c) Free shape recovery behaviour of SMP under different recovery temperatures (Tr).Tris taken as four different temperatures: 30, 35, 40 and 50 °C respectively. Full size image Figure 4a shows that the shape fixity can also be affected by the holding time at high temperatures. In Fig. 4a , after being held at T d for different time periods (6 × 10 0 s, 6 × 10 2 s and 6 × 10 3 s), all the samples were cooled to T L (20 °C) at the same cooling rate of 2.5 °C min −1 . Clearly, increasing the holding time improves the shape fixity. Therefore, combining Figs 3a and 4a , to achieve higher shape fixity, one can either increase the holding time or increase T d . This also inspires the postulation that different programming conditions, if designed well, could actually lead to the same shape fixity. Indeed, as indicated by the dashed line in the figure, the 90% shape fixity can be achieved by two programming conditions, T d =33.8 °C followed by stabilization at T d for 6 × 10 0 s and T d =30.0 °C followed by stabilization at T d for 6 × 10 2 s. Figure 4: Effects of holding time on Shape fixity and shape recovery. ( a ) Shape fixity as a function of programming temperature ( T d ) and holding time at T d . Note: dots denote the experimental results and solid lines denote simulation results the low temperature T L is always 20 °C in all the experimental cases. ( b ) Shape recovery behaviour of SMPs experienced by two programming conditions that achieve the same shape fix ratio (90%). ( c ) Free shape recovery behaviour of SMP under different recovery temperatures ( T r ). T r is taken as four different temperatures: 30, 35, 40 and 50 °C respectively. Full size image Since the two different programming conditions give to the same fixity, the next question is whether these two programming conditions lead to two different or identical recovery performances under the same recovery conditions. Figure 4b shows the experimental results of the above two cases ( T d =33.8 °C with 6 × 10 0 s holding time and T d =30.0 °C with 6 × 10 2 s holding time) by heating to T r (40 °C) at the heating rate of 2.5 °C min −1 . The corresponding shape recovery ratio is plotted in the figure as a function of heating time. The nearly overlapped shape recovery curves indicate that the same shape fixity will lead to the same recovery profile. Therefore, when the SMPs are subjected to the same free recovery condition, the shape recovery behaviour is essentially independent of the details of the programming history, but can be solely determined by the shape fixity. The influence of recovery condition on the free shape recovery behaviour of SMPs was evaluated by selecting different recovery temperatures ( T r =30° C, 35 °C, 40 °C and 50 °C respectively, Fig. 4c ) in the free recovery SM cycle. In these tests, the programming conditions were set identical with T d =40 °C and holding time of 6 × 10 2 s, which leads to a shape fixity of 98.7%. As shown in Fig. 4c , the recovery rate is faster at higher recovery temperatures. Note that for recovery temperatures greater than the glass transition temperature ( T g ) of SMPs (42.7 °C), the final shape recovery ratio is seen to be slightly larger than 100%. This is due to the thermal expansion for recovery temperatures greater than programming temperatures. The thermal expansion effect is neglected in the following discussions. A unified parameter: reduced time As shown above, the same fixity can be achieved by different programming methods and determines the free recovery. It then becomes intriguing to explore if there exists a parameter that determines the fixity and thus dictates the recovery. To answer this question, the analytical solution of the one-dimensional (1D) multi-branch rheological model was applied. Attempts were first made to examine the effectiveness of the model in capturing the experimental shape fixity of SMPs, following the same thermomechanical conditions in the experiments. The simulation results are presented in Fig. 4a and also compared with the experiments. It is seen that the 1D multi-branch rheological model successfully reproduced the experimental results. It should be noted that in the current experiment for the acrylate SMPs, the maximum stretch in each SM cycle is 20%. When large strain is applied (for example, up to 100%), polymer yielding behaviour might affect the model predictions and irrecoverable strain may occur in some polymer systems, which was addressed in recent work by Srinivasa et al. [61] , [62] . It is necessary to understand why different programming methods lead to the same fixity. For the above two mentioned programming conditions that lead to the same 90% shape fixity, the stress evolutions in each branch of the multi-branch model are plotted as histogram in Fig. 5 . When the SMP material is programmed at a lower temperature ( T d =30.0 °C, the second programming condition), the internal stress in each non-equilibrium branch is generally higher than that programmed at a higher temperature ( T d =33.8 °C, the first programming condition), especially in branches with small relaxation times. However, since the second programming condition has a longer holding time (6 × 10 2 s) at T d the amount of stress relaxation stress is higher. Therefore, the overall effect is that two programming conditions lead to the same internal stress state before and after the sudden unloading. 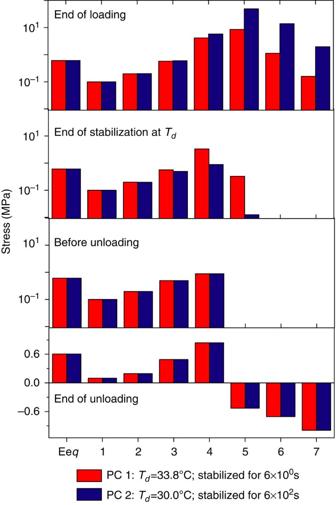Figure 5: Internal stress evolution in each branch of the multi-branch model. The two programming processes give the same shape fixity (90%). The number in thexaxis label denotes theith non-equilibrium branch. Figure 5: Internal stress evolution in each branch of the multi-branch model. The two programming processes give the same shape fixity (90%). The number in the x axis label denotes the i th non-equilibrium branch. Full size image Now we may conjecture that the same shape fixity is due to the same internal stress distribution before unloading. Indeed, this is confirmed by the calculation of R f based on the multi-branch modelling frame. During the sudden unloading, all the dashpots could be considered as frozen, and the shape fixity R f is calculated by the shape bouncing back, which can be calculated by the mechanical equilibrium (see Methods section): From Equation 5, since the denominator is a constant, the total stress before unloading dictates the shape fixity. To simplify the further analysis, we assume that the mechanical loading is instantaneous, and ignore the influence of thermal contraction on the rheological stress distribution under the constrained boundary condition. The effect of non-instantaneous loading conditions is discussed in Supplementary Note 2 . It is found that the influence of loading rate and thermal contraction is negligible in most SMP applications. The total stress before unloading can be therefore expressed as: where E relax ( t , T ) is the instantaneous relaxation modulus before unloading. Finally, Equation 7 also indicates that the instantaneous relaxation modulus before unloading determines the shape fixity of the SMP. It is well known that for thermo-rheologically simple polymers, the relaxation modulus follows the TTSP, that is where t r = α −1 ( T ) t ; α ( T ) is the shift factors in TTSP and is calculated using the method described in the Method section. Equation 8 states that the instantaneous relaxation modulus at temperature T after time t is equal to the relaxation modulus at temperature T 0 after time t r . For non-isothermal process, where t r is the reduced time [63] and t is the physical time during the experiments. Combining Equations 7, 8, 9, we have Equation 10 states that the reduced time t r measured at the reference temperature T 0 determines the shape fixity. In other words, if the two programming conditions have the same reduced programming time before unloading, they will lead to identical shape fixity. This is further confirmed by Table 1 , which lists the reduced time for the two programming conditions in Fig. 5 using T 0 =27.5 °C. Table 1 The reduced programming times before unloading in the two programming conditions that achieve the same shape fix ratio (90%). Full size table Since the relaxation modulus is a function of the reduced time, the reduced time is an effective measurement of the polymer rheological state during the programming process. As shown in Fig. 6 , three reduced times (1.0 × 10 3 s, 2.0 × 10 3 s and 3.0 × 10 3 s) are marked on the timing axis, and then respectively transferred back into the physical programming time according to the thermal history in the two programming conditions. The comparisons between the internal stress states show that the same reduced time, although corresponding to different physical times in the real programming conditions, leads to the same stress distribution in each branch of the model. Such a merit of reduced time provides theoretical basis to correlate alternative programming conditions to achieve the same fixity. 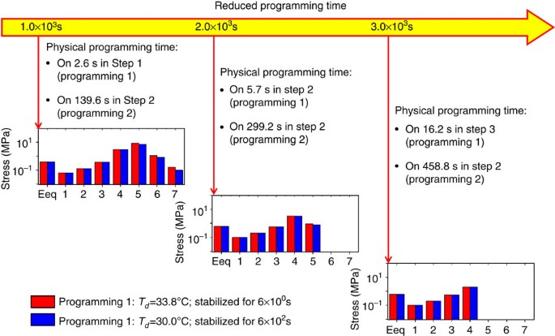Figure 6: Internal stress evlolution at different physical programming times. The same reduced programming time is mapped into two different programming conditions, showing the same internal stress distributions within branches. Figure 6: Internal stress evlolution at different physical programming times. The same reduced programming time is mapped into two different programming conditions, showing the same internal stress distributions within branches. Full size image In the following discussions, we demonstrate that the reduced time is also a unified parameter in predicting the free shape recovery of SMPs. In Fig. 7 , we replot Fig. 4c by transferring the physical time scale to the reduced time scale using Equation 9 with T 0 =27.5 °C. The four recovery curves at different recovery temperatures rejoin to form a master free recovery curve after the time scale transfer, which indicates that the free recovery behaviours of SMPs also follow the TTSP. According to the physical meaning of Equation 9, Fig. 7 also shows the recovery curve at T 0 =27.5 °C, which overlaps with the master free recovery curve obtained from the four free recovery curves. 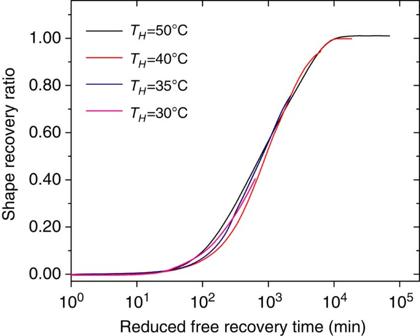Figure 7: Master free recovery curve. The four shape recovery curves presented inFig. 4cjoined to form a master free recovery curve after transferring the physical free recovery time into the reduced free recovery time. Figure 7: Master free recovery curve. The four shape recovery curves presented in Fig. 4c joined to form a master free recovery curve after transferring the physical free recovery time into the reduced free recovery time. Full size image The existence of the master free recovery curve inspires us to develop a method to predict their temperature-dependent free recovery behaviour. When the shape fixity is given, the stress distribution in each branch of the model before and after unloading can be obtained, which serves as the initial condition for the following free recovery process. Then using the analytical solutions to the multi-branch model under free recovery condition, the recovery ratio curves that correspond to different shape fixities are predicted at the reference temperature (27.5 °C) and shown in Fig. 8a . With different shape fixities, the SMP specimens recover at different rates and therefore different recovery ratios for a given recovery time. Then, by selecting R f =98.7% (the same as the above mentioned experimental results) recovery curve as the master curve, the time scale (actually represents the reduced free recovery time) is transferred back into different physical free recovery timing scales according to the specified thermal condition (heating to T r =30 °C, 35 °C, 40 °C and 50 °C, respectively) as illustrated in the experiments. Consequently, the temperature deponent free recovery curve is predicted in Fig. 8b . Comparisons between the simulation and experimental results presented in Fig. 8c indicate that the prediction method successfully captures the free recovery behaviours of the SMP at different recovery temperatures. 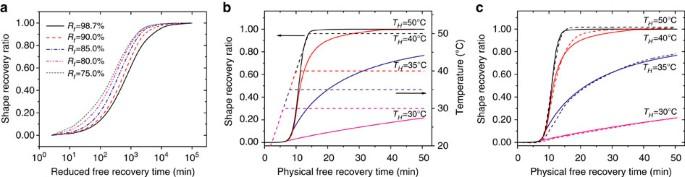Figure 8: Prediction on the shape recovery behaviour at different recovery temperatures. (a) The recovery temperature in each case is 27.5 °C while the programming temperature varies to achieve different shape fix ratio. Note: the 98.7% shape fixity represent the actual experimental results where the programming temperature is 40 °C. (b) SelectingRf=98.7% shape recovery curve as the master curve, then transfer the reduced time back into the real physical free recovery time according to the specified thermal condition (the dash lines represent the corresponding recovery temperatures). (c) Comparisons between the simulation and experimental results. The simulation curves are denoted as dash lines. Figure 8: Prediction on the shape recovery behaviour at different recovery temperatures. ( a ) The recovery temperature in each case is 27.5 °C while the programming temperature varies to achieve different shape fix ratio. Note: the 98.7% shape fixity represent the actual experimental results where the programming temperature is 40 °C. ( b ) Selecting R f =98.7% shape recovery curve as the master curve, then transfer the reduced time back into the real physical free recovery time according to the specified thermal condition (the dash lines represent the corresponding recovery temperatures). ( c ) Comparisons between the simulation and experimental results. The simulation curves are denoted as dash lines. Full size image The complicated dependence of polymer SM effect on the programming and free recovery conditions was unravelled by using the reduced time. Different thermo-temporal programming conditions can be measured by the reduced time at the reference temperature; the reduced time uniquely determines the shape fixity, which also uniquely determines the shape recovery in the reduced time scale. The free recovery in the physical time scale under different thermo-temporal conditions can be obtained by inversely converting the reduced time back into the physical time. This process inspires the creation of an SMP map shown in Fig. 9 . There are three quadrants in Fig. 9 . The bottom-left quadrant ( Fig. 9b ) shows the calculation of reduced programming time (the azimuthal direction) from holding time (the vertical axis) and programming temperatures (individual curves). The top-right quadrant ( Fig. 9c ) shows the conversion of the reduced recovery time (the vertical axis) to the physical recovery time (the vertical axis) at different temperatures (individual curves). The top-left quadrant ( Fig. 9a ) shows the fixity (the vertical axis on the left) as a function of reduced programming time by the white curve and the recovery ratio (represented by the contour colours) as a function of the reduced programming time and the reduced recovery time. 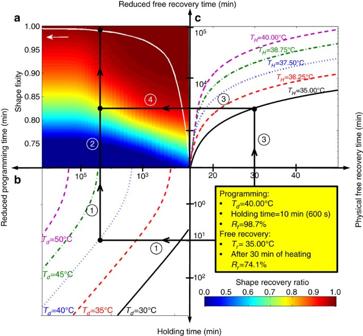Figure 9: The SM performance map. (a) A general referential contour. (b) Reduced programming time as a function of holding time and programming temperatureTd. (c) Reduced free recovery time as a function of heating temperatureTH. Note: other influencing factors are: loading rate=1% s−1; cooling rate=2.5 °C min−1;TL=20 °C; holding time atTL=1 h; heating rate=2.5 °C min−1. Figure 9: The SM performance map. ( a ) A general referential contour. ( b ) Reduced programming time as a function of holding time and programming temperature T d . ( c ) Reduced free recovery time as a function of heating temperature T H . Note: other influencing factors are: loading rate=1% s −1 ; cooling rate=2.5 °C min −1 ; T L =20 °C; holding time at T L =1 h; heating rate=2.5 °C min −1 . Full size image To use the SMP map, one starts with using the bottom-left quadrant to obtain the reduced programming time from a programming temperature and a holding time. With the reduced programming time, one then obtains the fixity from the white curve in the top-left quadrant. For a given recovery condition (with a recovery temperature and the time at that temperature), one obtains the reduced recovery time from the top-right quadrant. Then finally, using the reduced programming time and the reduced recovery time, one obtains the recovery ratio from the contour in the top-left quadrant. Fig. 9 also shows an example with a specified programming and free recovery condition. Assuming that the programming temperature T d =40 °C, holding time at T d =10 min, the reduced programming time (2.30 × 10 4 min) is determined by following Path 1 in Fig. 9b , which further pinpoints the shape fixity (98.7%) by following Path 2 in Fig. 9a . For the subsequent free recovery step, if the intended recovery temperature T r =35 °C and the total heating time is 30 min, the reduced recovery time is determined by Path 3 in Fig. 9c . Using this reduced recovery time, together with the reduced programming time, we obtain the recovery ratio (contour) as 74.1% (Path 4 in Fig. 9a ). The SMP map also shows the general trend of the effects of programming conditions and recovery conditions on fixity and recovery ratio. For example, for a given programming temperature, a longer holding time leads to a longer reduced programming time, and therefore a higher shape fixity. Also, a longer reduced recovery time leads to a higher recovery ratio. Finally, for a given reduced recovery time, a shorter programming time leads to a higher recovery ratio, but at the price of a lower shape fixity. As will be shown in the next section and Supplementary Note 3 , the SMP map can be readily constructed using the simple multi-branch model, whose parameters can be determined by stress relaxation experiments and a DMA test, which are standard rheological tests in polymer physics. Therefore, the SMP map can be constructed from the standard polymer rheological experiments. However, it should be noted that the study in this paper is based on SMPs that are thermo-rheologically simple and achieve their SM effects through glass transition. For other types of SMPs, such as those due to crystallization, it is unclear if the proposed theory can be applied. In addition, for the two materials studied in this paper, an acrylate-based SMP and an epoxy-based SMP (results shown in Supplementary Note 3 ), we showed small strain dynamic mechanical analysis can provide a good estimation of SM behaviours of the SMPs for the programming strain up to the intermediate strain level (20% for the acrylate SMP and 60% for the epoxy SMP). However, cautions should be taken if a polymer demonstrates a highly nonlinear or inelastic behaviour. For example, the SMP based on thermoplastic polyurethane [64] , [65] , [66] , [67] can present a yielding behaviour at the strain of 5–20% and exhibit permanent set after unloading [68] . Small strain dynamic mechanical analysis cannot provide a thorough characterization of the thermoviscoelastic (or thermoviscoplastic) behaviours and thus may not be able to provide an accurate estimation of the SM performance. In this case, nonlinear modelling approach, such as those presented recently by Srinivasa et al. [61] , [62] can be used. Material and experiments The SMP material used in this study was an acrylate-based network polymer. Its liquid monomer tert-butyl acrylate (tBA), liquid crosslinker poly (ethylene glycol) dimethacrylate (PEGDMA) and the photo polymerization initiator (2,2-dimethoxy-2-phenylacetophenone) in powder form were ordered from Aldrich and used in their as received conditions without any further purification. The synthesis procedure of the SMP followed Yakacki et al. [31] by mixing the tBA monomer, crosslinker and photo polymerization initiator with a weight ratio of 4,000:1,000:1, and the solution was then exposed to UV irradiation for 10 min before the final heat treatment at 90 °C for 1 h to assist the complete conversion of monomers. All the experiments involved in this paper were conducted on a Dynamic Mechanical Analyzer (DMA, TA Instruments, Model Q800) in the tensile mode. The SMP was cast into rectangular specimens with a uniform dimension of 10 mm × 3 mm × 0.2 mm. Multi-branch rheological model Considering the thermomechanical deformations experienced by the SMP materials during the above mentioned experimental demonstrations, we briefly introduce the analytical solutions to the viscous response of the applied model under (1) strain controlled loading condition and (2) free recovery condition. In a strain controlled loading condition, the strain evolution in each branch is independent. Assuming e m is the strain in the equilibrium branch, is the elastic strains in the i th nonequilibrium branch. Owing to the series arrangement of the spring and the dashpot in a Maxwell element, the requirement of identical stress in these two elements yields where τ i is the temperature-dependent relaxation time in each nonequilibrium branch, and can be calculated by the well-established ‘thermorheological simplicity’ principle [58] : where α T ( T ) is the time–temperature superposition shifting factor. is the reference relaxation time at the reference temperature T s . For temperatures above and near T s , shifting factors follow the classic Williams–Landel–Ferry (WLF) equation [69] : where C 1 and C 2 are material constants. T M is the WLF reference temperature. For temperatures below T s , shifting factors follow the Arrhenius-type behaviour [70] : where A is a material constant, F c is the configurational energy and k b is Boltzmann’s constant. The total stress evolution of the model is then expressed as the summation of each branch: During the free recovery process, the strain evolution in each branch is highly coupled and could not be solved individually. Since there is no force applied to the specimen, the total stress is zero during the free recovery, Then, we can write the system governing equations in the matrix form: or with [ A ]=[ E ] −1 [ T ], [ E ] ij = E j / E eq +δ ij and [ T ] ij =δ ij / , where δ ij is the Kronecker Delta, [ e e ] i = and respectively denote the strain and strain changing rate of different nonequilibrium branches. The system governing Equation 18 was solved by diagonalizing [ A ] by using its modal matrix [ Q ]: where λ i is the i-th eigenvalue of matrix [ A ], . By further examining Equation 19, we can tell that the evolution of is only dependent on the physical recovery time t and the shift factor α ( T ). According to the definition of reduced time (Eq. 9), we have: where t r is the reduced time and T 0 is the reference temperature. From the analytical point of view, this expression explains why the free recovery behaviour of SMPs follows the time–temperature superposition. In view of the obtained , we can push it back to by , and then derive the total strain evolution: Shape fixity Before unloading, the total stress is given by Equation 1. After unloading, and the material recovers recover by a small amount of strain Δ e . Therefore, the fixity is Since the total stress is zero, we have Therefore, Note that the numerator in the above equation is also the total stress before unloading, we obtain Equation 5. Determination of model parameters The parameters for the multi-branch model are determined by using the TTSP-based stress relaxation tests on the acrylate SMPs. Detailed experimental procedure and results can be found in the Supplementary Note 1 . The determined model parameters are listed in Table 2 . Table 2 Parameters of the developed constitutive model. Full size table In Table 2 , the glass transition temperature T g (42.7 °C) is determined by using the DMA tests. The WLF reference temperature T M is typically 10–15 °C below T g . The parameters in WLF and Arrhenius equations are determined during the shifting of relaxation curves into the master curve. T s is calculated by equating α T inEquations 12 and 13. The number of nonequilibrium branches, the relaxation time in each nonequilibrium branch and the elastic modulus of each spring are determined by fitting the stress relaxation master curve (see Supplementary Note 1 for details). How to cite this article: Yu, K. et al. Reduced time as a unified parameter determining fixity and free recovery of shape memory polymers. Nat. Commun. 5:3066 doi: 10.1038/ncomms4066 (2014).